Highly self-reactive naive CD4 T cells are prone to differentiate into regulatory T cells Upon activation, naive CD4 T cells differentiate into a variety of T-helper-cell subsets characterized by different cytokine production and functions. Currently, lineage commitment is considered to depend mostly on the environmental context to which naive CD4 T cells are exposed. Here we challenge this model based on the supposed homogeneity of the naive CD4 T-cell compartment. We show that peripheral naive CD4 T cells can be subdivided into two subsets according to Ly-6C expression. Furthermore, the two newly defined subsets (Ly-6C − and Ly-6C + naive CD4 T cells) are not equal in their intrinsic ability to commit into the induced regulatory T-cell lineage. Finally, phenotypic analysis, imaging and adoptive transfer experiments reveal that Ly-6C expression is modulated by self-recognition, allowing the dichotomization of the naive CD4 T-cell compartment into two cell subsets with distinct self-reactivity. Altogether, our results show that naive CD4 T cells with the highest avidity for self are prone to differentiate into regulatory T cells. In normal young adult mice, the peripheral CD4 T-cell compartment is composed of almost 80% naive T cells. The remaining 20% are distributed between regulatory and effector/memory-phenotype CD4 T cells. Following activation by antigen-presenting cells (APCs) in the periphery, naive CD4 T (CD4 T N ) cells can differentiate into a variety of well-documented T-helper (T H ) cell subsets, such as T H 1, T H 2, T H 17 or induced regulatory T (iTreg) cells, characterized by their cytokine-production profiles and specific effector functions. For instance, T H 1 cells are characterized by their production of interferon (IFN)-γ, a potent activator of cell-mediated immunity [1] , [2] . T H 2 cells are characterized by production of interleukin (IL)-4, IL-5 and IL-13, which are potent activators of B-cell immunoglobulin production [1] , [2] . In addition, T H 17 cells are characterized by IL-17A, IL-17F and IL-22 secretion and are described to have an important role in anti-microbial responses [3] , [4] . Finally, iTreg cells produce transforming growth factor-β (TGF-β) and share phenotypic and functional characteristics with natural regulatory T cells that have a crucial role in maintaining peripheral self-tolerance [5] . Identification of T-bet, GATA-3, RORγt/RORα and Foxp3 as lineage-defining transcription factors solidified the categorization into T H 1, T H 2, T H 17 and iTreg effector cell subsets [6] , [7] , [8] , [9] , [10] . Additional T H cell subsets have also been described, such as IL-10 producing type 1 regulatory T cells [11] , IL-9 producing T H 9 cells [12] or T FH cells [13] . Lineage commitment leads to a broad diversity of effector cell functions and is considered to depend mostly on the immunological context in which CD4 T N cells are immersed at the time of their activation. Indeed, the differentiation fate appears predominantly governed by extrinsic factors such as cytokines or environmental cues. Specifically, in vitro culture assays and in vivo models have been used to establish that IL-12, IL-4, TGF-β alone or TGF-β in combination with pro-inflammatory cytokines, such as IL-6, are crucially required for T H 1, T H 2, iTreg or T H 17-cell differentiation, respectively [14] , [15] , [16] , [17] , [18] . This commonly accepted model implicitly posits that the CD4 T N cells on which the various cytokines act constitute an homogeneous population of cells. However, intrinsic heterogeneity within the CD4 T N -cell pool such as TCR affinity for antigen or sensitivity to co-stimulatory signals and cytokines should be taken into account when considering, in vivo , CD4 T N -cell differentiation [19] . In light of these considerations, we decided to study whether intrinsic properties of CD4 T N cells, in association with the cytokine environment in which they are immersed, could contribute to helper CD4 T-cell commitment. Here we show that peripheral CD4 T N cells can be subdivided into two subsets according to Ly-6C expression. These two newly defined subsets are not equal in their intrinsic ability to commit into the iTreg-cell lineage with Ly-6C − CD4 T N cells differentiating more efficiently into iTreg cells than their Ly-6C + -cell counterparts both in vivo and in vitro . Heterogeneity of Ly-6C expression in CD4 T N cells Throughout this study, CD4 T N lymphocytes were defined as Foxp3 − CD25 − CD44 − /lo CD4 + CD8α − TCRβ + cells ( Supplementary Fig. S1a ). Although the CD4 T N -cell compartment is commonly considered as homogenous, we observed, as previously described [20] , [21] , that CD4 T N cells from the secondary lymphoid organs of C57BL/6 mice (peripheral lymph node (pLN) and mesenteric lymph node (mLN) and spleen) can be subdivided into two subsets according to Ly-6C expression ( Fig. 1a,b ). This applied also to CD4 T N cells from bone marrow (BM), Peyer’s patches, blood and peritoneal cavity. Although the proportion of CD4 T N cells varied greatly between these organs, in all of them, about two-thirds of CD4 T N cells expressed Ly-6C ( Supplementary Fig. S1b ). In contrast, Ly-6C + CD4 T N cells were almost completely absent in the thymus. 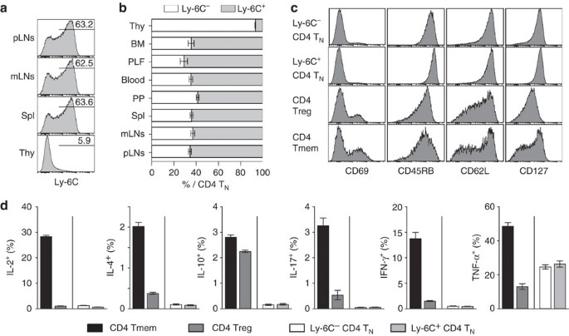Figure 1: CD4 TNcells can be subdivided into two subsets on the basis of Ly-6C molecule expression. (a) Ly-6C fluorescence histograms of CD4 TNcells (CD4+CD8α−TCRβ+Foxp3−CD25−CD44−/loT cells) recovered from pLNs, mLNs, spleen (Spl) and thymus (Thy) are shown for a representative C57BL/6 Foxp3-GFP mouse. Numbers in each histogram represent the percentage of Ly-6C+cells among CD4 TNcells. (b) The proportions of Ly-6C−and Ly-6C+cells among CD4 TNcells recovered from the thymus, BM, peritoneal lavage fluid (PLF), blood, Peyer’s patches (PP), spleen, mLNs and pLNs of C57BL/6 mice were calculated. Results are shown as means±s.e.m. for six mice from two independent experiments. (c) CD69, CD45RB, CD62L and CD127 fluorescence histograms of pLN Ly-6C−CD4 TNcells, Ly-6C+CD4 TNcells, regulatory CD4 T cells (CD4 Treg defined as Foxp3+CD4+CD8α−TCRβ+) and memory CD4 T cells (CD4 Tmem defined as Foxp3−CD44hiCD4+CD8α−TCRβ+cells) are shown for a representative C57BL/6 Foxp3-GFP mouse. The histograms are representative of at least six mice from three individual experiments. (d) The proportions of IL-2, IL-4, IL-10, IL-17, IFN-γ or TNF-α producing cells among memory, regulatory, Ly-6C−and naive Ly-6C+CD4 TNcells recovered from pLNs of C57BL/6 Foxp3-GFP mice were estimated after a pulse stimulation with phorbol myristate acetate and ionomycin. Results are shown as means±s.e.m. for six mice from two independent experiments. Figure 1: CD4 T N cells can be subdivided into two subsets on the basis of Ly-6C molecule expression. ( a ) Ly-6C fluorescence histograms of CD4 T N cells (CD4 + CD8α − TCRβ + Foxp3 − CD25 − CD44 − /lo T cells) recovered from pLNs, mLNs, spleen (Spl) and thymus (Thy) are shown for a representative C57BL/6 Foxp3-GFP mouse. Numbers in each histogram represent the percentage of Ly-6C + cells among CD4 T N cells. ( b ) The proportions of Ly-6C − and Ly-6C + cells among CD4 T N cells recovered from the thymus, BM, peritoneal lavage fluid (PLF), blood, Peyer’s patches (PP), spleen, mLNs and pLNs of C57BL/6 mice were calculated. Results are shown as means±s.e.m. for six mice from two independent experiments. ( c ) CD69, CD45RB, CD62L and CD127 fluorescence histograms of pLN Ly-6C − CD4 T N cells, Ly-6C + CD4 T N cells, regulatory CD4 T cells (CD4 Treg defined as Foxp3 + CD4 + CD8α − TCRβ + ) and memory CD4 T cells (CD4 Tmem defined as Foxp3 − CD44 hi CD4 + CD8α − TCRβ + cells) are shown for a representative C57BL/6 Foxp3-GFP mouse. The histograms are representative of at least six mice from three individual experiments. ( d ) The proportions of IL-2, IL-4, IL-10, IL-17, IFN-γ or TNF-α producing cells among memory, regulatory, Ly-6C − and naive Ly-6C + CD4 T N cells recovered from pLNs of C57BL/6 Foxp3-GFP mice were estimated after a pulse stimulation with phorbol myristate acetate and ionomycin. Results are shown as means±s.e.m. for six mice from two independent experiments. Full size image Both Ly-6C − and Ly-6C + CD4 T N cells from pLNs exhibited a true naive phenotype illustrated by their high expression of CD45RB, CD62L and CD127 and their lack of expression of CD69 ( Fig. 1c ). Consistent with their naive phenotype, both T N -cell subsets were not able to produce IL-2, IL-4, IL-10, IL-17 or IFN-γ in response to stimulation ( Fig. 1d ). By contrast, memory-phenotype CD4 T cells (CD4 Tmem cells) produced all of these cytokines and, as expected, regulatory CD4 T cells (CD4 Treg cells) synthesized IL-10. Finally, we observed that a similar proportion of Ly-6C − and Ly-6C + CD4 T N cells produced TNF-α. Therefore, Ly-6C expression divides the peripheral CD4 T N -cell compartment into two subsets. Pathogenicity of Ly-6C − and Ly-6C + CD4 T N cells To test whether the phenotypic heterogeneity of the CD4 T N -cell compartment might reveal differential expansion/differentiation potentials, highly purified Ly-6C − or Ly-6C + CD4 T N cells were transferred into T-cell-deficient recipients ( Fig. 2a , Supplementary Fig. S2 ). T-cell compromised animals injected with CD4 T N cells are known to rapidly develop inflammatory bowel disease (IBD) [22] , [23] . Interestingly, mice injected with Ly-6C − CD4 T N cells developed with time a more severe wasting disease than those injected with Ly-6C + CD4 T N cells ( Fig. 2b ). This correlated with higher histological colitis scores (determined 7 weeks after transfer by examination of colon sections) when mice were injected with Ly-6C − CD4 T N cells ( Fig. 2c ). Surprisingly, contrasting with clinical observations, Ly-6C − CD4 T N cells expanded to a lesser extent than their Ly-6C + -cell counterparts when transferred into T-cell-deficient recipients ( Fig. 2d ). Differences were not only quantitative as, in all studied secondary lymphoid organs, Ly-6C − CD4 T N cells gave rise to greater proportions and absolute numbers of iTreg cells as compared with Ly-6C + CD4 T N cells ( Fig. 2e , Supplementary Fig. S3 ). In addition, although Ly-6C + CD4 T N -cell transfer led to higher proportions and absolute numbers of IFNγ-producing CD4 T cells in secondary lymphoid organs, the differentiation of Ly-6C − CD4 T N cells resulted in greater proportions and absolute numbers of newly generated IL-17 + CD4 T cells ( Fig. 2f , Supplementary Fig. S3 ). Interestingly, the proportion of IL-17 + CD4 T cells was tightly correlated with the proportion of newly generated iTreg cells ( Fig. 2g ). These latter results suggest that, in the IBD experimental model, iTreg-cell generation promotes T H 17 CD4 T-cell development as recently suggested in other settings [24] , [25] . 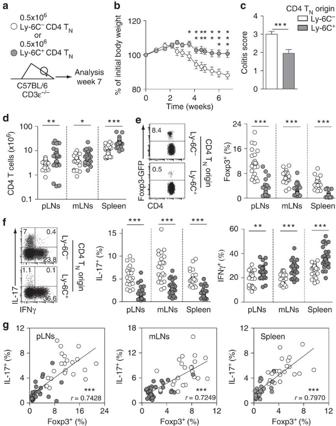Figure 2: Differential pathogenicity of Ly-6C−and Ly-6C+CD4 TNcells after transfer into T-cell-deficient recipients. 0.5 × 106flow-cytometry-sorted Ly-6C−or Ly-6C+CD4 TNcells from C57BL/6 Foxp3-GFP mice were injected intravenously into C57BL/6 CD3ε−/−mice. Seven weeks after transfer, pLNs, mLNs and spleen were recovered separately. (a) Diagram illustrating the experimental model. (b) Body weight of recipient mice was monitored up to 7 weeks post transfer, and percentages of initial body weight were calculated and plotted. (c) Colitis scores of recipient mice were assessed 7 weeks after transfer. (d) Absolute numbers of CD4 T cells recovered from pLNs, mLNs and spleen of recipient mice. (e) Foxp3-GFP/CD4 dot-plots for gated CD4+CD8α−CD3+T cells recovered from pLNs of representative recipient mice and proportion of Foxp3+cells among CD4+CD8α−CD3+T cells recovered from pLNs, mLNs and spleen of recipient mice. (f) IL-17/IFNγ dot-plots for gated CD4+CD8α−CD3+T cells recovered from pLNs of representative recipient mice and proportion of IL-17- and IFNγ-producing CD4+CD8α−CD3+T cells recovered from pLNs, mLNs and spleen of recipient mice. (g) Correlation between the proportion of Foxp3-expressing and IL-17-producing cells among CD4+CD8α−CD3+T cells recovered from pLNs, mLNs and spleen of recipient mice. (b–c) Results are shown as means±s.e.m. for at least six mice per group per experiment, from four independent experiments. (d–g) Each dot represents an individual mouse. (b–f) Significance of differences between two series of results was assessed using a two-tailed unpaired Student’st-test. (g) Correlation analyses were performed using Pearson’s correlation test. Values ofP<0.05 were considered as statistically significant (*P<0.05; **P<0.01; and ***P<0.001). Figure 2: Differential pathogenicity of Ly-6C − and Ly-6C + CD4 T N cells after transfer into T-cell-deficient recipients. 0.5 × 10 6 flow-cytometry-sorted Ly-6C − or Ly-6C + CD4 T N cells from C57BL/6 Foxp3-GFP mice were injected intravenously into C57BL/6 CD3ε − / − mice. Seven weeks after transfer, pLNs, mLNs and spleen were recovered separately. ( a ) Diagram illustrating the experimental model. ( b ) Body weight of recipient mice was monitored up to 7 weeks post transfer, and percentages of initial body weight were calculated and plotted. ( c ) Colitis scores of recipient mice were assessed 7 weeks after transfer. ( d ) Absolute numbers of CD4 T cells recovered from pLNs, mLNs and spleen of recipient mice. ( e ) Foxp3-GFP/CD4 dot-plots for gated CD4 + CD8α − CD3 + T cells recovered from pLNs of representative recipient mice and proportion of Foxp3 + cells among CD4 + CD8α − CD3 + T cells recovered from pLNs, mLNs and spleen of recipient mice. ( f ) IL-17/IFNγ dot-plots for gated CD4 + CD8α − CD3 + T cells recovered from pLNs of representative recipient mice and proportion of IL-17- and IFNγ-producing CD4 + CD8α − CD3 + T cells recovered from pLNs, mLNs and spleen of recipient mice. ( g ) Correlation between the proportion of Foxp3-expressing and IL-17-producing cells among CD4 + CD8α − CD3 + T cells recovered from pLNs, mLNs and spleen of recipient mice. ( b – c ) Results are shown as means±s.e.m. for at least six mice per group per experiment, from four independent experiments. ( d – g ) Each dot represents an individual mouse. ( b – f ) Significance of differences between two series of results was assessed using a two-tailed unpaired Student’s t -test. ( g ) Correlation analyses were performed using Pearson’s correlation test. Values of P <0.05 were considered as statistically significant (* P <0.05; ** P <0.01; and *** P <0.001). Full size image iTreg cells promote T H 17 differentiation in an IBD model We then performed co-transfer experiments in which Ly-6C − CD4 T N cells from CD45.2 mice were co-injected with Ly-6C + CD4 T N cells from CD45.1 mice into T-cell-deficient recipients ( Fig. 3a ). T-cell-deficient mice injected with Ly-6C − or Ly-6C + CD4 T N cells alone were used in parallel as control mice ( Supplementary Fig. S4a ). 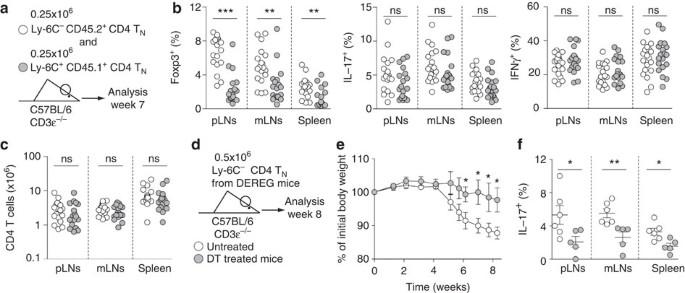Figure 3: Newly generated iTreg cells promote TH17-cell differentiation after CD4 TN-cell transfer into T-cell-deficient recipients. (a–c) Ly-6C−CD4 TNcells (0.25 × 106) from C57BL/6 Foxp3-GFP CD45.2 mice were injected intravenously (i.v.) into C57BL/6 CD3ε−/−mice together with 0.25 × 106Ly-6C+CD4 TNcells from C57BL/6 Foxp3-GFP CD45.1 mice. Seven weeks after transfer, pLNs, mLNs and spleen were recovered separately and analysed. (a) Diagram illustrating the experimental model. (b) Proportions of CD45.1+or CD45.2+CD4 T cells expressing Foxp3 or producing IL-17 or IFNγ recovered from pLNs, mLNs and spleen of recipient mice. (c) Absolute numbers of CD45.1+or CD45.2+CD4 T cells recovered from pLNs, mLNs and spleen of recipient mice. (d–f) Ly-6C−CD4 TNcells (0.5 × 106) from DEREG mice were injected i.v. into C57BL/6 CD3ε−/−mice treated or not twice a week with DT. (d) Diagram illustrating the experimental model. (e) Body weight of recipient mice was monitored up to 8 weeks post transfer, and percentages of initial body weight were calculated and plotted. (f) Proportions of IL-17-producing CD4+CD8α−CD3+T cells recovered from pLNs, mLNs and spleen of recipient mice. (b,c,f) Each dot represents an individual mouse. (e,f) Results are shown as means±s.e.m. for two independent experiments. Significance of differences between two series of results was assessed using a two-tailed paired (b,c) or unpaired (e,f) Student’st-test. Values ofP<0.05 were considered as statistically significant (*P<0.05; **P<0.01; and ***P<0.001). ns, not significant. Figure 3: Newly generated iTreg cells promote T H 17-cell differentiation after CD4 T N -cell transfer into T-cell-deficient recipients. ( a – c ) Ly-6C − CD4 T N cells (0.25 × 10 6 ) from C57BL/6 Foxp3-GFP CD45.2 mice were injected intravenously (i.v.) into C57BL/6 CD3ε − / − mice together with 0.25 × 10 6 Ly-6C + CD4 T N cells from C57BL/6 Foxp3-GFP CD45.1 mice. Seven weeks after transfer, pLNs, mLNs and spleen were recovered separately and analysed. ( a ) Diagram illustrating the experimental model. ( b ) Proportions of CD45.1 + or CD45.2 + CD4 T cells expressing Foxp3 or producing IL-17 or IFNγ recovered from pLNs, mLNs and spleen of recipient mice. ( c ) Absolute numbers of CD45.1 + or CD45.2 + CD4 T cells recovered from pLNs, mLNs and spleen of recipient mice. ( d – f ) Ly-6C − CD4 T N cells (0.5 × 10 6 ) from DEREG mice were injected i.v. into C57BL/6 CD3ε − / − mice treated or not twice a week with DT. ( d ) Diagram illustrating the experimental model. ( e ) Body weight of recipient mice was monitored up to 8 weeks post transfer, and percentages of initial body weight were calculated and plotted. ( f ) Proportions of IL-17-producing CD4 + CD8α − CD3 + T cells recovered from pLNs, mLNs and spleen of recipient mice. ( b , c , f ) Each dot represents an individual mouse. ( e , f ) Results are shown as means±s.e.m. for two independent experiments. Significance of differences between two series of results was assessed using a two-tailed paired ( b , c ) or unpaired ( e , f ) Student’s t -test. Values of P <0.05 were considered as statistically significant (* P <0.05; ** P <0.01; and *** P <0.001). ns, not significant. Full size image Mice co-injected with both Ly-6C − and Ly-6C + CD4 T N cells developed a wasting disease and colitis as severe as mice injected with Ly-6C − CD4 T N cells alone ( Supplementary Fig. S4b,c ). When both cell subsets were injected together, Ly-6C − CD4 T N cells still gave rise to a higher proportion of newly differentiated iTreg cells than their Ly-6C + -cell counterparts ( Fig. 3b ). By contrast, in all secondary lymphoid organs studied, neither expansion nor T H 17/T H 1 differentiation appeared significantly different between both transferred cell subsets ( Fig. 3b,c ). More precisely, when injected together, Ly-6C − and Ly-6C + CD4 T N cells gave rise to proportions of IL-17 + among CD4 T cells similar to those observed when Ly-6C − CD4 T N cells were injected alone ( Supplementary Fig. S5 ). We then analysed, in this setting, the correlations between the ability of Ly-6C − CD4 T N cells to differentiate into iTreg cells and the capacity of co-injected Ly-6C − and Ly-6C + CD4 T N cells to give rise to IL-17-producing CD4 T cells ( Supplementary Fig. S6 ). Interestingly, the proportion of IL-17-producing CD4 T cells arising from initially injected Ly-6C − (CD45.2) and Ly-6C + (CD45.1) CD4 T N cells similarly correlated with the percentage of iTreg cells generated from CD45.2 + Ly-6C − CD4 T N cells. These results agreed with our hypothesis that newly differentiated iTreg cells would favour T H 17-cell differentiation. Finally, we conducted iTreg-cell-depletion experiments. Ly-6C − CD4 T N cells from DEREG mice [26] were injected into T-cell-deficient recipients treated or not with diphtheria toxin (DT) twice a week ( Fig. 3d ). As expected, DT efficiently depleted iTreg cells ( Supplementary Fig. S7a,b ). More interestingly, DT treatment resulted in the reduction of the severity of the wasting disease ( Fig. 3e ) correlated with a significant decrease of the histological colitis score ( Supplementary Fig. S7c ). Depletion of iTreg cells also led to a strong inhibition of T H 17-cell development ( Fig. 3f ). Taken together, our data strongly suggest that, in our experimental model, iTreg-cell differentiation promotes T H 17-cell generation. Efficient Ly-6C- CD4 TN-cell polarization into iTreg cells Ly-6C − CD4 T N cells were more efficient in differentiating into iTreg cells than Ly-6C + CD4 T N cells in vivo when transferred into a lymphopenic environment. To further assess whether this characteristic feature was an intrinsic property of Ly-6C − CD4 T N cells, we performed iTreg-cell polarization assays in vitro . Purified Ly-6C − or Ly-6C + CD4 T N cells were stimulated with anti-CD3- and anti-CD28-coated antibodies (Abs) in the presence of graded doses of TGFβ. Although they expressed similar amounts of the TGFβ receptors I and II ( Supplementary Fig. S8 ), Ly-6C − CD4 T N cells gave rise to a twofold higher proportion of iTreg cells than Ly-6C + CD4 T N cells did for suboptimal doses of exogenous TGFβ ( Fig. 4a ). Differences were quantitative rather than qualitative, as iTregs cells generated from both Ly-6C − and Ly-6C + CD4 T N cells displayed similar suppressive capacities ( Fig. 4b ). Two groups have recently described that suboptimal activation of CD4 T N cells in the absence of exogenous TGFβ led to their conversion into iTreg cells [27] , [28] . In this setting, a more efficient conversion was also observed in Ly-6C − CD4 T N -cell cultures ( Supplementary Fig. S9 ). 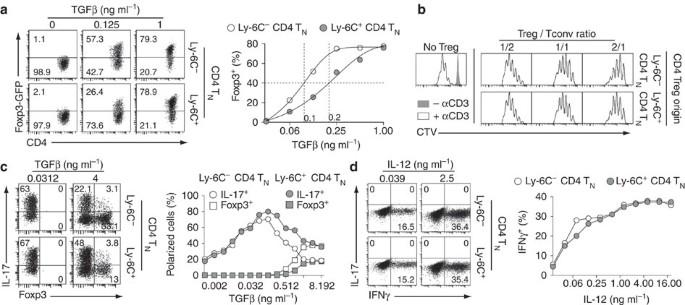Figure 4: Ly-6C−CD4 TNcells differentiate more efficiently into iTreg cells than Ly-6C+CD4 TNcellsin vitro. (a) Purified LN Ly-6C−or Ly-6C+CD4 TNcells from C57BL/6 Foxp3-GFP mice were stimulated for 4 days with coated anti-CD3 and anti-CD28 Abs in the presence of graded concentrations of TGFβ1. Representative Foxp3-GFP/CD4 dot-plots for gated CD4 T cells and the proportion of Foxp3+cells among CD4 T cells are shown as a function of TGFβ1 concentration. (b) Purified Ly-6C−or Ly-6C+CD4 TNcells were stimulated for 3 days with coated anti-CD3 and anti-CD28 Abs in the presence of 1 ng ml−1of TGFβ1 and then let to rest for 3 more days in the presence of IL-2 (13 ng ml−1). GFP-expressing cells were then sorted using flow cytometry, and their suppressive abilities to inhibit the proliferation of Cell Trace Violet-labelled conventional CD4 T cells (LN GFP−CD4 T cells from C57BL/6 Foxp3-GFP mice) in response to anti-CD3 Abs in the presence of APCs were tested. (c) Ly-6C−or Ly-6C+CD4 TNcells from C57BL/6 Foxp3-GFP mice were stimulated for 4 days with coated anti-CD3 and anti-CD28 Abs in the presence of IL-6 (20 ng ml−1) and graded concentrations of TGFβ1. Representative IL-17/Foxp3 dot-plots for gated CD4 T cells, the proportion of IL-17-producing CD4 T cells and the proportion of Foxp3+cells among CD4 T cells are shown as a function of TGFβ1 concentration. (d) Ly-6C−or Ly-6C+CD4 TNcells from C57BL/6 Foxp3-GFP mice were stimulated for 4 days with coated anti-CD3 and anti-CD28 Abs in the presence of graded concentrations of IL-12. Representative IL-17/IFNγ dot-plots for gated CD4 T cells and the proportion of IFNγ-producing CD4 T cells are shown as a function of IL-12 concentration. Results are representative of at least three independent experiments. Figure 4: Ly-6C − CD4 T N cells differentiate more efficiently into iTreg cells than Ly-6C + CD4 T N cells in vitro . ( a ) Purified LN Ly-6C − or Ly-6C + CD4 T N cells from C57BL/6 Foxp3-GFP mice were stimulated for 4 days with coated anti-CD3 and anti-CD28 Abs in the presence of graded concentrations of TGFβ1. Representative Foxp3-GFP/CD4 dot-plots for gated CD4 T cells and the proportion of Foxp3 + cells among CD4 T cells are shown as a function of TGFβ1 concentration. ( b ) Purified Ly-6C − or Ly-6C + CD4 T N cells were stimulated for 3 days with coated anti-CD3 and anti-CD28 Abs in the presence of 1 ng ml −1 of TGFβ1 and then let to rest for 3 more days in the presence of IL-2 (13 ng ml −1 ). GFP-expressing cells were then sorted using flow cytometry, and their suppressive abilities to inhibit the proliferation of Cell Trace Violet-labelled conventional CD4 T cells (LN GFP − CD4 T cells from C57BL/6 Foxp3-GFP mice) in response to anti-CD3 Abs in the presence of APCs were tested. ( c ) Ly-6C − or Ly-6C + CD4 T N cells from C57BL/6 Foxp3-GFP mice were stimulated for 4 days with coated anti-CD3 and anti-CD28 Abs in the presence of IL-6 (20 ng ml −1 ) and graded concentrations of TGFβ1. Representative IL-17/Foxp3 dot-plots for gated CD4 T cells, the proportion of IL-17-producing CD4 T cells and the proportion of Foxp3 + cells among CD4 T cells are shown as a function of TGFβ1 concentration. ( d ) Ly-6C − or Ly-6C + CD4 T N cells from C57BL/6 Foxp3-GFP mice were stimulated for 4 days with coated anti-CD3 and anti-CD28 Abs in the presence of graded concentrations of IL-12. Representative IL-17/IFNγ dot-plots for gated CD4 T cells and the proportion of IFNγ-producing CD4 T cells are shown as a function of IL-12 concentration. Results are representative of at least three independent experiments. Full size image We then compared the capacity of Ly-6C − and Ly-6C + CD4 T N cells to polarize into T H 1 and T H 17 cells in vitro ( Fig. 4c,d ). In response to low doses of TGFβ in the presence of IL-6, Ly-6C − and Ly-6C + CD4 T N cells gave rise to similar proportions of T H 17 cells. However, for high doses of TGFβ, Ly-6C − CD4 T N cells differentiated less efficiently into T H 17 cells than their Ly-6C + -cell counterparts ( Fig. 4c ). This decreased ability of Ly-6C − CD4 T N cells to generate T H 17 cells in response to high doses of TGFβ may derive from the fact that part of them differentiated into iTreg cells in these conditions despite the presence of IL-6. CD4 T N -cell polarization into T H 1 cells did not differ whether or not cells were initially expressing Ly-6C ( Fig. 4d ). Taken together, our data strongly suggest that Ly-6C − CD4 T N cells have an intrinsic higher capacity to differentiate into iTreg cells than their Ly-6C + -cell counterparts, whereas both subsets differentiate with a similar efficiency into T H 1 and T H 17 cells. Ly-6C expression is acquired in the periphery We then decided to determine where and when Ly-6C expression was acquired by CD4 T N cells. To follow thymic output and specifically identify recent thymic emigrants in secondary lymphoid organs, we used recombination-activating gene 2 promoter (RAG2p)-green fluorescent protein (GFP) transgenic mice, in which GFP expression is driven by the RAG2p. The transgene generates a bright GFP signal during thymic differentiation that remains detectable in the periphery throughout the first few days after their migration [29] . Although most CD4 T N single-positive thymocytes were Ly-6C − , about 40% of CD4 T N recent thymic emigrants (GFP hi ) in LNs already expressed Ly-6C molecule, suggesting that the acquisition of Ly-6C expression by CD4 T N cells occurs very rapidly after their exit from the thymus ( Fig. 5a ). Furthermore, the proportion of Ly-6C + cells among peripheral CD4 T N lymphocytes increased with GFP brightness decay, indicating that acquisition of Ly-6C expression occurred in a rapid and gradual manner over time. 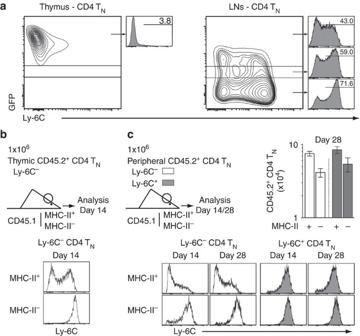Figure 5: Ontogeny of Ly-6C−and Ly-6C+CD4 TNcells. (a) GFP/Ly-6C contour plots and Ly-6C fluorescence histograms of gated CD4 TNcells recovered from the thymus and LNs of a representative C57BL/6 RAG2p-GFP reporter mouse. Numbers in each histogram represent the percentage of Ly-6C+cells among the indicated CD4 TNcell subsets. (b) 1 × 106thymic Ly-6C−CD4 TNcells from C57BL/6 Foxp3-GFP CD45.2 mice were injected intravenously (i.v.) into C57BL/6 CD45.1 mice lacking (MHC-II−) or not lacking (MHC-II+) MHC class II molecule expression. A diagram illustrating the experimental model and Ly-6C fluorescence histograms of gated CD45.2+CD4 TNcells recovered from LNs of recipient mice 14 days after transfer are shown. (c) Ly-6C−(1 × 106) or Ly-6C+CD4 TNcells from LNs of C57BL/6 Foxp3-GFP CD45.2 mice were injected i.v. into CD45.1 C57BL/6 mice lacking or not lacking MHC class II molecule expression. A diagram illustrating the experimental model is shown. The absolute numbers of CD45.2+CD4 TNcells recovered from the periphery (LNs+spleen) of recipient mice 28 days after transfer are shown as means±s.e.m. Ly-6C fluorescence histograms of CD45.2+CD4 TNcells recovered from LNs of recipient mice 14 and 28 days after transfer are shown. Results are representative of at least two independent experiments. Figure 5: Ontogeny of Ly-6C − and Ly-6C + CD4 T N cells. ( a ) GFP/Ly-6C contour plots and Ly-6C fluorescence histograms of gated CD4 T N cells recovered from the thymus and LNs of a representative C57BL/6 RAG2p-GFP reporter mouse. Numbers in each histogram represent the percentage of Ly-6C + cells among the indicated CD4 T N cell subsets. ( b ) 1 × 10 6 thymic Ly-6C − CD4 T N cells from C57BL/6 Foxp3-GFP CD45.2 mice were injected intravenously (i.v.) into C57BL/6 CD45.1 mice lacking (MHC-II − ) or not lacking (MHC-II + ) MHC class II molecule expression. A diagram illustrating the experimental model and Ly-6C fluorescence histograms of gated CD45.2 + CD4 T N cells recovered from LNs of recipient mice 14 days after transfer are shown. ( c ) Ly-6C − (1 × 10 6 ) or Ly-6C + CD4 T N cells from LNs of C57BL/6 Foxp3-GFP CD45.2 mice were injected i.v. into CD45.1 C57BL/6 mice lacking or not lacking MHC class II molecule expression. A diagram illustrating the experimental model is shown. The absolute numbers of CD45.2 + CD4 T N cells recovered from the periphery (LNs+spleen) of recipient mice 28 days after transfer are shown as means±s.e.m. Ly-6C fluorescence histograms of CD45.2 + CD4 T N cells recovered from LNs of recipient mice 14 and 28 days after transfer are shown. Results are representative of at least two independent experiments. Full size image Then, we injected Ly-6C − CD4 T N single-positive thymocytes from CD45.2 mice into CD45.1 mice expressing or lacking major histocompatibility complex (MHC) class II molecules ( Fig. 5b ). As expected, Ly-6C − CD4 T N single-positive thymocytes gave rise to both Ly-6C − and Ly-6C + CD4 T N cells after transfer into MHC class II-competent recipients. More surprisingly, all CD45.2 + CD4 T N cells recovered from MHC class II-deficient recipients were expressing Ly-6C, suggesting that all CD4 T N cells acquired Ly-6C expression or that survival of Ly-6C − CD4 T N cells was highly compromised in this context. To address these issues, peripheral Ly-6C − or Ly-6C + CD4 T N cells from CD45.2 mice were transferred into CD45.1 mice expressing or lacking MHC class II molecules ( Fig. 5c ). The survival of both Ly-6C − and Ly-6C + CD45.2 + CD4 T N -cell subsets was affected by MHC class II molecule deprivation, excluding the hypothesis of a preferential disappearance of Ly-6C − CD4 T N cells in MHC class II-deficient recipients. Ly-6C expression by CD45.2 + CD4 T N cells was also assessed. First, we noticed that Ly-6C − and Ly-6C + phenotypes were rather stable over time after transfer into MHC class II-competent recipients. One can notice that some CD4 T N cells, initially Ly-6C − , expressed low levels of this marker 14 days after transfer. However, this percentage remained relatively stable thereafter (33.1±2.1 on day 14 versus 37.3±1.9 on day 28, not significant). By contrast, virtually all peripheral CD45.2 + CD4 T N cells recovered from MHC class II-deficient recipients expressed Ly-6C whether or not they were expressing it before transfer. One may argue that MHC class II-deficient recipients lack not only MHC class II molecule expression but also endogenous CD4 T cells and that this latter point introduces another element of variability between both types of recipients. To address this issue, we generated BM chimeras in which CD4 T cells were produced in the thymus but were unable to interact with MHC class II molecules in the periphery ( Supplementary Fig. S10a (refs 30 , 31 )). Although such chimeras contained as many peripheral CD4 T cells as control chimeras 4 weeks after BM cell transfer, almost all their CD4 T N cells were expressing Ly-6C in the periphery ( Supplementary Fig. S10b, c ). Altogether, these results suggest that the downmodulation of Ly-6C expression by CD4 T N cells is dependent on continuous interactions with MHC class II molecules. Ly-6C expression is modulated by self-recognition In line with a role for TCR signalling in the modulation of Ly-6C expression in CD4 T N cells, we found that in vitro Ly-6C + CD4 T N -cell activation in response to TCR stimulation led to Ly-6C downregulation ( Supplementary Fig. S11 ). Injection of CD4 T N cells into lymphopenic recipients (such as in the IBD model) led to the activation, the strong proliferation and the conversion into memory-like cells of part of the injected cells in response to self and environmental antigens, a process known as spontaneous proliferation [32] , [33] . This CD4 T-cell spontaneous proliferation relied on interactions with MHC class II molecules, and 2 weeks after transfer, most CD4 T cells recovered from the periphery of recipient mice derived from this process. Interestingly, the progeny of both Ly-6C − or Ly-6C + CD4 T N cells was lacking Ly-6C expression 2 weeks after transfer into lymphopenic recipients ( Supplementary Fig. S12 ). Thus, the TCR signals leading to T-cell activation induced Ly-6C downregulation both in vitro and in vivo . We hypothesized that Ly-6C surface levels on CD4 T N cells might predict their propensity to interact with peripheral self-MHC class II molecules and thus to receive subthreshold TCR signals. CD5 expression on CD4 T N cells has been shown to be adjusted to reflect TCR contact with self [34] , [35] , [36] , [37] . In fact, the more a CD4 T N cell interacts with self, the more this cell expresses CD5. We thus analysed the expression of CD5, but also of CD4 and of the TCR itself by peripheral Ly-6C − and Ly-6C + CD4 T N cells. Consistent with our hypothesis, we observed that Ly-6C − CD4 T N cells exhibited significantly higher densities of CD5 and lower levels of the TCRβ chain and CD4 compared with their Ly-6C + -cell counterparts ( Fig. 6a ). Mandl et al. [37] have recently shown that the more CD4 T N cells expressed CD5, the more the ζ-chain of the CD3 complex was phosphorylated. In line with a higher capacity of Ly-6C − CD4 T N cells to interact with self, we found that the extent of CD3ζ phosphorylation was far more important in Ly-6C − CD4 T N cells than in Ly-6C + CD4 T N cells (pζ/ζ ratio, Fig. 6b and Supplementary Fig. S11 ). 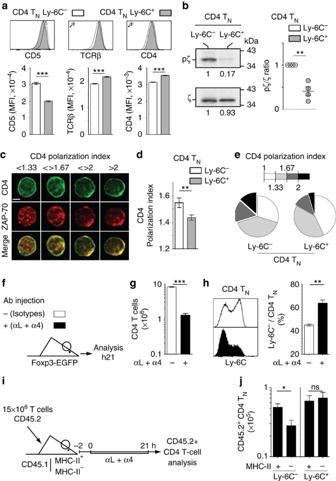Figure 6: Ly-6C−CD4 TNcells continuously interact with MHC class II molecules. (a) CD5, TCRβ and CD4 fluorescence histograms of gated Ly-6C−and Ly-6C+CD4 TNcells from LNs of a representative C57BL/6 Foxp3-GFP mouse. Mean fluorescence intensities (MFIs) are shown as means±s.e.m. for at least six mice from two independent experiments. (b) Flow-cytometry-sorted Ly-6C−and Ly-6C+CD4 TNcells (3 × 105cells/condition) were lysed, and both CD3ζ protein levels (ζ) and the extent of CD3ζ chain phosphorylation (pζ) were determined by immunoblotting. The pζ/ζ ratio was then quantified. Each dot represents an individual sample. (c,d) LN cells from C57BL/6 Foxp3-GFP mice were fixed immediately in 4% paraformaldehyde after isolation. Ly-6C−or Ly-6C+CD4 TNcells were then purified and stained for CD4 (green) and ZAP-70 (red) expression. (c) Representative CD4 and ZAP-70 sum-projection images are shown. Scale bar, 5 μm. (d) CD4 polarization indexes were estimated for Ly-6C−(n=212) or Ly-6C+(n=352) CD4 TNcells by automated analyses of two independent experiments (see Methods). (e) Distribution of Ly-6C−or Ly-6C+CD4 TNcells as a function of their CD4 polarization index. (f–h) C57BL/6 Foxp3-GFP mice were injected or not intraperitoneally with anti-αL and anti-α4 Abs to block LN entry. Twenty-one hours later, LNs were recovered and CD4 T cells were analysed. (f) Diagram illustrating the experimental model. (g) Absolute numbers of CD4 T cells in mLNs. (h) Representative Ly-6C fluorescence histograms and percentages of Ly-6C−cells are shown for CD4 TNcells recovered from mLNs of treated and untreated mice. (i–j) T cells (15 × 106) from CD45.2 C57BL/6 Foxp3-GFP mice were transferred into C57BL/6 CD45.1 mice lacking (MHC-II−) or not lacking (MHC-II+) MHC class II molecule expression. Two hours later, LN entry was blocked. LNs were collected 21 h after entry blockade, and CD45.2+CD4 T cells were analysed. (i) Diagram illustrating the experimental model. (j) Absolute numbers of CD45.2+CD4 T cells in mLNs. Results are representative of at least two independent experiments. Significance of differences between two series of results was assessed using a two-tailed paired (b) or unpaired (d,g,h,j) Student’st-test. Values ofP<0.05 were considered as statistically significant (*P<0.05; **P<0.01; and ***P<0.001). ns, not significant. Figure 6: Ly-6C − CD4 T N cells continuously interact with MHC class II molecules. ( a ) CD5, TCRβ and CD4 fluorescence histograms of gated Ly-6C − and Ly-6C + CD4 T N cells from LNs of a representative C57BL/6 Foxp3-GFP mouse. Mean fluorescence intensities (MFIs) are shown as means±s.e.m. for at least six mice from two independent experiments. ( b ) Flow-cytometry-sorted Ly-6C − and Ly-6C + CD4 T N cells (3 × 10 5 cells/condition) were lysed, and both CD3ζ protein levels (ζ) and the extent of CD3ζ chain phosphorylation (pζ) were determined by immunoblotting. The pζ/ζ ratio was then quantified. Each dot represents an individual sample. ( c , d ) LN cells from C57BL/6 Foxp3-GFP mice were fixed immediately in 4% paraformaldehyde after isolation. Ly-6C − or Ly-6C + CD4 T N cells were then purified and stained for CD4 (green) and ZAP-70 (red) expression. ( c ) Representative CD4 and ZAP-70 sum-projection images are shown. Scale bar, 5 μm. ( d ) CD4 polarization indexes were estimated for Ly-6C − ( n =212) or Ly-6C + ( n =352) CD4 T N cells by automated analyses of two independent experiments (see Methods). ( e ) Distribution of Ly-6C − or Ly-6C + CD4 T N cells as a function of their CD4 polarization index. ( f – h ) C57BL/6 Foxp3-GFP mice were injected or not intraperitoneally with anti-αL and anti-α4 Abs to block LN entry. Twenty-one hours later, LNs were recovered and CD4 T cells were analysed. ( f ) Diagram illustrating the experimental model. ( g ) Absolute numbers of CD4 T cells in mLNs. ( h ) Representative Ly-6C fluorescence histograms and percentages of Ly-6C − cells are shown for CD4 T N cells recovered from mLNs of treated and untreated mice. ( i – j ) T cells (15 × 10 6 ) from CD45.2 C57BL/6 Foxp3-GFP mice were transferred into C57BL/6 CD45.1 mice lacking (MHC-II − ) or not lacking (MHC-II + ) MHC class II molecule expression. Two hours later, LN entry was blocked. LNs were collected 21 h after entry blockade, and CD45.2 + CD4 T cells were analysed. ( i ) Diagram illustrating the experimental model. ( j ) Absolute numbers of CD45.2 + CD4 T cells in mLNs. Results are representative of at least two independent experiments. Significance of differences between two series of results was assessed using a two-tailed paired ( b ) or unpaired ( d , g , h , j ) Student’s t -test. Values of P <0.05 were considered as statistically significant (* P <0.05; ** P <0.01; and *** P <0.001). ns, not significant. Full size image We then decided to image Ly-6C − and Ly-6C + CD4 T N cells. Stefanova et al. [38] have shown that recognition of self-ligands by CD4 T N cells induced the clustering of the TCR complex and associated signalling molecules to the region of the lymphocyte membrane in contact with APCs. Here we found that LN CD4 T N cells directly fixed after isolation exhibited various degrees of clustering of both the CD4 co-receptor and ZAP-70 ( Fig. 6c ). We quantified CD4 polarization and found that the CD4 polarization index was significantly greater in Ly-6C − CD4 T N cells than in Ly-6C + CD4 T N cells ( Fig. 6d ). More precisely, Ly-6C − CD4 T N cells contained a higher proportion of cells exhibiting high degree of CD4 polarization than their Ly-6C + -cell counterparts ( Fig. 6e ). Thus, at one given time, a higher proportion of Ly-6C − than Ly-6C + CD4 T N cells might be interacting with APCs in LNs. A greater ability of Ly-6C − CD4 T N cells to interact with self-MHC class II molecules should have consequences on their behaviour in secondary lymphoid organs. Mandl et al. [36] have recently shown that interactions with MHC class II molecules retained CD4 T N cells in LNs. By using the same protocol ( Fig. 6f ), we analysed the phenotype of CD4 T N cells remaining within LNs after entry blockade. Most CD4 T cells have egressed from LNs 21 h after entry blockade ( Fig. 6g ). Interestingly, Ly-6C − cells were greatly enriched in the remaining CD4 T N cells ( Fig. 6h ). We then verified that retention of Ly-6C − CD4 T N cells in LNs after entry blockade was due to interactions with MHC class II molecules. To do so, we injected CD45.2 + T cells into CD45.1 recipients lacking (MHC-II − ) or expressing (MHC-II + ) MHC class II molecules. Two hours later, LN entry was blocked and LNs were collected 21 h after entry blockade ( Fig. 6i ). Although the absolute numbers of remaining Ly-6C + CD4 T N cells were unaffected by MHC class II deprivation, those of Ly-6C − CD4 T N cells were significantly decreased in recipients lacking MHC class II molecules ( Fig. 6j ). This was not due to the acquisition of Ly-6C expression by Ly-6C − CD4 T N cells, as 24 h were not sufficient to induce upregulation of this marker ( Supplementary Fig. S13 ). Thus, interactions with MHC class II molecules only retained Ly-6C − CD4 T N cells within LNs. These last results are in line with the greater average polarization of CD4 and ZAP-70 molecules at the cell surface of Ly-6C − CD4 T N cells and suggest that Ly-6C − CD4 T N cells are interacting more strongly than Ly-6C + CD4 T N cells with MHC class II-expressing cells in peripheral secondary lymphoid organs. Self-recognition reinforces iTreg-cell differentiation We then determined whether self-recognition might have a role in the differential ability of Ly-6C − and Ly-6C + CD4 T N cells to differentiate into iTreg cells. First, we studied the expression of CD5 and Ly-6C by peripheral monoclonal CD4 T N cells from AND and Marylin TCR-transgenic mice in a RAG2 − / − background. It has recently been shown that AND CD4 T cells have a higher avidity for self than Marylin CD4 T cells [37] , [39] , [40] . Indeed, AND CD4 T cells expressed far higher density of CD5 than Marylin CD4 T cells ( Fig. 7a (ref. 37 )). In agreement with our assumption that Ly-6C non-expression might reflect the magnitude of CD4 T N -cell self-reactivity, all Marylin CD4 T cells were expressing high surface amounts of Ly-6C, whereas the majority of AND CD4 T cells did not ( Fig. 7a ). Finally, in line with our experiments with polyclonal CD4 T N cells, we observed that AND CD4 T cells differentiated far more efficiently than Marilyn CD4 T cells into iTreg cells in vitro ( Fig. 7b ). 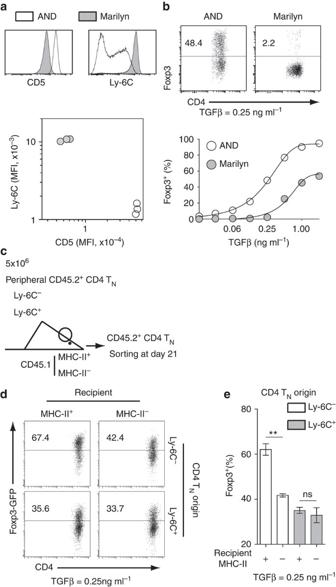Figure 7: Self-recognition reinforces the ability of CD4 TNcells to differentiate into iTreg cells. (a) CD5 and Ly-6C fluorescence histograms and graph representing Ly-6C MFI of gated CD4 TNcells from LNs of AND (solid line/white) and Marylin (filled histogram/grey) TCR-transgenic mice as a function of their CD5 MFI. Each dot represents an individual mouse. (b) CD4 TNcells from LNs of AND and Marylin TCR-transgenic mice were stimulated for 4 days with coated anti-CD3 and anti-CD28 Abs in the presence of graded concentrations of TGFβ1. Representative Foxp3/CD4 dot-plots for gated CD4 T cells and the proportion of Foxp3+cells among CD4 T cells are shown as a function of TGFβ1 concentration. (c–e) Ly-6C−(5 × 106) or Ly-6C+CD4 TNcells from LNs of C57BL/6 Foxp3-GFP CD45.2 mice were injected i.v. into CD45.1 C57BL/6 mice lacking or not lacking MHC class II molecule expression (MHC-II−and MHC-II+, respectively). CD45.2+CD4 TNcells were then FACS-sorted 21 days after transfer from the periphery of recipient mice and stimulated for 4 days with coated anti-CD3 and anti-CD28 Abs in the presence of 0.25 ng ml−1of TGFβ1. (c) Diagram illustrating the experimental model. (d) Representative Foxp3-GFP/CD4 dot-plots for gated CD4 T cells are shown as a function of recipient mice and CD4 TN-cell origin. (e) Proportion of Foxp3+cells among CD4 T cells as a function of recipient mice and CD4 TNcells origin are shown as means±s.e.m. for at least six mice from two independent experiments. Significance of differences between two series of results was assessed using a two-tailed unpaired Student’st-test. Values ofP<0.05 were considered as statistically significant (**P<0.01). ns, not significant. Figure 7: Self-recognition reinforces the ability of CD4 T N cells to differentiate into iTreg cells. ( a ) CD5 and Ly-6C fluorescence histograms and graph representing Ly-6C MFI of gated CD4 T N cells from LNs of AND (solid line/white) and Marylin (filled histogram/grey) TCR-transgenic mice as a function of their CD5 MFI. Each dot represents an individual mouse. ( b ) CD4 T N cells from LNs of AND and Marylin TCR-transgenic mice were stimulated for 4 days with coated anti-CD3 and anti-CD28 Abs in the presence of graded concentrations of TGFβ1. Representative Foxp3/CD4 dot-plots for gated CD4 T cells and the proportion of Foxp3 + cells among CD4 T cells are shown as a function of TGFβ1 concentration. ( c – e ) Ly-6C − (5 × 10 6 ) or Ly-6C + CD4 T N cells from LNs of C57BL/6 Foxp3-GFP CD45.2 mice were injected i.v. into CD45.1 C57BL/6 mice lacking or not lacking MHC class II molecule expression (MHC-II − and MHC-II + , respectively). CD45.2 + CD4 T N cells were then FACS-sorted 21 days after transfer from the periphery of recipient mice and stimulated for 4 days with coated anti-CD3 and anti-CD28 Abs in the presence of 0.25 ng ml −1 of TGFβ1. ( c ) Diagram illustrating the experimental model. ( d ) Representative Foxp3-GFP/CD4 dot-plots for gated CD4 T cells are shown as a function of recipient mice and CD4 T N -cell origin. ( e ) Proportion of Foxp3 + cells among CD4 T cells as a function of recipient mice and CD4 T N cells origin are shown as means±s.e.m. for at least six mice from two independent experiments. Significance of differences between two series of results was assessed using a two-tailed unpaired Student’s t -test. Values of P <0.05 were considered as statistically significant (** P <0.01). ns, not significant. Full size image Second, we adoptively transferred Ly-6C − and Ly-6C + CD4 T N cells from CD45.2 mice into CD45.1 recipients expressing or lacking MHC class II molecules ( Fig. 7c ). Three weeks after transfer, CD45.2 + CD4 T N cells were purified from the periphery of recipient mice and assessed for their ability to differentiate into iTreg cells in vitro . For suboptimal doses of TGFβ, cells purified from MHC-II-competent recipients initially injected with Ly-6C − CD4 T N cells gave rise to a twofold higher proportion of iTreg cells than cells derived from MHC class II-deficient recipients initially injected with the same cells or from MHC-II-competent recipients initially injected with Ly-6C + CD4 T N cells ( Fig. 7d,e ). Altogether, our data strongly suggest that the ability of a naive T cell to commit into the iTreg-cell lineage pathway upon in vitro stimulation is shaped by its capacity to interact with self in its original environment. Over the last decades, the CD4 T N cells have been commonly considered as a homogenous T-cell compartment. In the present paper, we confirm that Ly-6C expression splits this compartment into positive and negative cells with one-third of peripheral CD4 T cells lacking this marker [20] , [21] . Expression of Ly-6C is acquired in the periphery as almost all thymocytes are Ly-6C − . More precisely, analysis of RAG2p-GFP mice and adoptive transfer experiments indicate that thymocytes rapidly gain Ly-6C expression upon migration to the periphery. Then, the expression of Ly-6C by peripheral CD4 T N cells is stable over time. Moreover, several lines of evidence strongly suggest that the expression of Ly-6C by peripheral CD4 T N cells inversely correlates with their ability to interact with self. First, all thymic and peripheral CD4 T N cells gained Ly-6C expression when transferred into MHC class II-deficient recipients. Second, Ly-6C − CD4 T N cells expressed more CD5 and exhibited a higher degree of CD3ζ phosphorylation than Ly-6C + CD4 T N cells. Third, Ly-6C − CD4 T N cells exhibit a higher degree of co-clustering of the CD4 co-receptor and the TCR-associated signalling molecule, ZAP-70, than their Ly-6C + -cell counterparts. Finally, interactions with MHC class II molecules retained preferentially Ly-6C − CD4 T N cells within LNs, therefore increasing their transit time. Thus, altogether, our data indicate that Ly-6C − CD4 T N cells are more ‘autoreactive’ than their Ly-6C + -cell counterparts. Repeated subthreshold TCR stimulations are triggered within secondary lymphoid organs where T cells interact with self-peptides while scanning the surface of dendritic cells. Stefanova et al. [38] have first shown that interruption of CD4 T N -cell contact with self leads to a rapid decline on signalling and response sensitivity to foreign stimuli. These data were further confirmed by several elegant studies and shown to apply also to CD8 T N cells [41] , [42] , [43] . Recently, using CD5 expression to discriminate between T N cells interacting strongly (CD5 hi ) or not (CD5 lo ) with self, several groups have shown that TCR contact with self in the periphery causes CD8 T N cells to be hypersensitive to IL-2, IL-7 and IL-15 (refs 44 , 45 , 46 ). Altogether, these results strongly suggest that self-recognition not only allows the survival of T N cells but also increase quantitatively their responsiveness towards their cognate antigens for both CD4 and CD8 T N cells, and towards ILs in the case of CD8 T N cells [47] . However, it has not been yet addressed whether self-recognition qualitatively affects the response of T N cells to stimulation. Here we propose that the ability of a CD4 T N cell to differentiate into an iTreg cell upon apropriate stimulation would be shaped by self-reactivity. In line with this assumption, Ly-6C − CD4 T N cells that are likely to interact strongly with MHC class II molecule-expressing cells in LNs are the cells that differentiate more efficiently into iTreg cells both in vitro and in vivo . Moreover, disruption of interactions with MHC class II molecules decreases the commitment efficacy of Ly-6C − CD4 T N cells towards the iTreg-cell lineage. Indeed, the iTreg-cell polarization potential of Ly-6C − CD4 T N cells parked for 3 weeks in MHC class II-deficient recipients dropped to the level observed in Ly-6C + CD4 T N cells, the potential of which is not affected by MHC deprivation. Thus, self-recognition may affect not only quantitatively but also qualitatively the response of CD4 T N cells to their cognate antigens. Upon activation, a CD4 T N cell can differentiate into a great variety of effector cells including T H 1, T H 2, T H 17 or iTreg cells. The present paradigm assumes that the choice made by CD4 T N cells to commit into one of these lineages would be mainly governed by extrinsic factors with an important role of the cytokines released in the environment at the time of their activation. Several data, including those presented here, extend this theory by showing that intrinsic factors also have a role in CD4 T N -cell fate determination. Fifteen years ago, several studies have proposed that the strength of the TCR signal at the time of antigen recognition would have a role in the T H 1/T H 2 lineage choice [48] , [49] . More recently, Gottschalk et al. [50] have shown that a low dose of a strong agonist resulted in maximal induction of iTreg cells. Thus, differentiation of CD4 T N cells into iTreg cells upon stimulation relies not only on extrinsic factors such as the presence of TGFβ in their environment but also on intrinsic factors such as the avidity of the TCR, which they express for both self and foreign ligands. Altogether, our results strongly suggest that CD4 T N cells with the highest avidity for self (Ly-6C − CD4 T N cells) have a biased commitment towards the iTreg-cell lineage and that this intrinsic ability is linked to their enhanced pathogenicity when injected into lymphopenic mice. Indeed, colitis in mice transferred with Ly-6C − CD4 T N cells is prevented if Tregs are depleted. This last result may appear paradoxical, given the vast literature showing that Tregs prevent colitis in lymphopenic mice when co-transferred together with CD4 T N cells. The nature of Tregs by itself (natural versus induced Tregs), their number (iTregs represent from 4.7 to 11.4% of the CD4 T cells recovered from the secondary lymphoid organs of recipient mice at the end point of our experiments, whereas when co-injected at a physiological rate together with CD4 T N cells (one Treg for eight CD4 T N cells), they represent >25% of expanding peripheral CD4 T cells as soon as 1 week after transfer [51] ) or the timing of the presence of Tregs in the periphery (from the beginning when co-transferred together with CD4 T N cells versus the time required for their generation and expansion in our setting) may explain these opposite effects of Tregs in the IBD experimental model. In other settings, in particular in lymphoreplete animals, an enhanced ability of the most autoreactive CD4 T N cells to commit to the iTreg-cell lineage pathway might represent a previously undescribed mechanism of self-tolerance. This process would diminish the risk of the most self-reactive CD4 T cells to become deleterious effector cells through responding to bacteria, viruses or parasites. Indeed, such a mechanism would allow the organism to augment its own protection during each infectious episode, especially by avoiding molecular mimics to induce novel, potent and self-peptide-reactive CD4 T-cell effectors when T-cell responses raised against the pathogen cross-react with self-peptides. Mice C57BL/6 mice (CD45.2) were obtained from Charles River Laboratories. C57BL/6 CD45.1, C57BL/6 CD3ε − / − , C57BL/6 MHC-II Δ/Δ CD45.1 and C57BL/6 AND TCR-transgenic RAG2 − / − mice were maintained in our own animal facilities, under specific pathogen-free conditions. C57BL/6 Marilyn TCR-transgenic RAG2 − / − mice were provided by Dr Emmanuel Donnadieu, Institut Cochin, Paris, France. C57BL/6 Foxp3-GFP CD45.2 [52] and C57BL/6 DEREG [26] mice were initially obtained from Dr Bernard Malissen, Centre d'Immunologie de Marseille-Luminy, France, and Dr Tim Sparwasser, Institute of Infection Immunology, TWINCORE, Hannover, Germany, respectively. C57BL/6 Foxp3-GFP CD45.2 mice were then crossed with C57BL/6 CD45.1 mice to generate C57BL/6 Foxp3-GFP CD45.1 mice. C57BL/6 RAG2p-GFP reporter mice [53] were provided by Dr Antonio Bandeira, Unité du Développement des Lymphocytes, Institut Pasteur, Paris, France. Four- to 12-week-old mice were used for all experiments. Donor and recipient mice were sex-matched. Experiments were carried out in accordance with the guidelines of the French Veterinary Department. All procedures performed were approved by the Paris-Descartes Ethical Committee for Animal Experimentation (decision CEEA34.CA.080.12). Cell suspensions pLNs, mLNs, spleen and thymus were homogenized and passed through a nylon cell strainer (BD Falcon) in RPMI 1640 Glutamax (Gibco) supplemented with 10% FCS (Biochrom) for adoptive transfer (LNs only), or in 5% FCS and 0.1% NaN 3 (Sigma-Aldrich) in PBS for flow cytometry. Adoptive transfer of CD4 T N cells CD4 T cells were purified from LNs (pooled superficial cervical, axillary, brachial, inguinal and mLNs) or thymi of C57BL/6 Foxp3-GFP or DEREG mice by incubating cell suspensions on ice for 20 min with a mixture of anti-CD8 (53-6.7), anti-CD11b (Mac-1) and anti-CD19 (1D3) Abs obtained from hybridoma supernatants, and then with magnetic beads coupled to anti-rat immunoglobulins (Dynal Biotech). Purified CD4 T cells were then labelled with biotinylated anti-Ly-6C (AL-21), PE-conjugated anti-CD25 (PC61), APC-conjugated anti-CD44 (IM7), all from BD Biosciences, and Pacific Blue-conjugated streptavidin (Invitrogen). Ly-6C − and Ly-6C + CD4 T N cells were sorted as GFP − CD25 − CD44 − /lo cells using a FACS-ARIA3 flow cytometer (BD Biosciences) and injected intravenously into sex-matched recipient mice. In the experiments depicted in Fig. 3d–f and Supplementary Fig. 7 , recipient mice were injected intraperitoneally 2 consecutive days per week with 500 ng of DT (Sigma-Aldrich). Adoptive transfer of BM cells BM cells were incubated on ice for 20 min with anti-CD4 (GK1.5) and anti-CD8 a (53-6.7) Abs, obtained from hybridoma supernatants, and then with magnetic beads coupled to anti-rat immunoglobulin (Dynal Biotech). We injected 5 × 10 6 T-cell-depleted BM cells intravenously into each lethally irradiated (9.5 Gy) recipient mouse. Cell surface staining and flow cytometry Cell suspensions were collected and dispensed into 96-well round-bottom microtiter plates (Greiner Bioscience; 6 × 10 6 cells per well). Surface staining was performed by incubating the cells on ice, for 15 min per step, with Abs in 5% FCS (Biochrom) and 0.1% NaN 3 (Sigma-Aldrich) PBS. Each cell-staining reaction was preceded by a 15-min incubation with a purified anti-mouse CD16/32 Ab (FcγRII/III block; 2.4G2) obtained from hybridoma supernatants. For determination of intracellular cytokine production, cells were stimulated with 0.5 μg ml −1 phorbol myristate acetate (Sigma-Aldrich), 0.5 μg ml −1 ionomycin (Sigma-Aldrich) and 10 μg ml −1 Brefeldin A (Sigma-Aldrich) for 2 h at 37 °C. Cells were then stained for surface markers, fixed in 2% paraformaldehyde in PBS and permeabilized with 0.5% saponin, followed by labelling with specific cytokine Abs. PerCP-conjugated anti-CD4 (RM4-5), phycoerythrin (PE)-conjugated anti-CD5 (53-7.3), anti-CD25 (PC61), anti-CD45.1 (A20), anti-CD69 (H1.2F3), anti-TCRβ (H57-597), anti-IL-2 (JES6-5H4), anti-IL-4 (11B11), anti-IL-10 (JES5-16E3) and anti-IL-17A (TC11-18H10), APC-conjugated anti-CD44 (IM7), anti-TCRβ (H57-597), anti-IFN-γ (XMG1.2), streptavidin, fluorescein isothiocyanate-conjugated anti-TNF-α (MP6-XT22), PE-Cy7-conjugated anti-Ly-6C (AL-21), streptavidin, PerCP-Cy5.5-conjugated anti-CD45.2 (104), APC-H7-conjugated anti-CD8 (53-6.7), Pacific Blue-conjugated anti-CD4 (RM4-5), and Alexa Fluor 700-conjugated anti-Ly-6C (AL-21), biotinylated anti-Ly-6C (AL-21), anti-CD5 (53-6.7), anti-CD45.1 (A20), anti-CD45.2 (104), anti-CD45RB (16A) and anti-CD62L (MEL14) were obtained from BD Biosciences. PE-conjugated anti-CD45.2 (104), PE-Cy5-conjugated anti-CD25 (PC61.5), Alexa Fluor 700-conjugated anti-CD45.2 (104), PerCP-Cy5.5-conjugated anti-TCRβ (H57-597) and biotinylated anti-CD127 (A7R34) were obtained from eBioscience. Pacific Blue-conjugated streptavidin was obtained from Invitrogen. Multi-colour immunofluorescence was analysed using a BD-LSR2 cytometer (BD Biosciences). List-mode data files were analysed using Diva software (BD Biosciences). Data acquisition and cell sorting were performed on the Cochin Immunobiology facility. Immunoblot analysis Ly-6C − and Ly-6C + CD4 T N cells (3 × 10 5 cells per condition) were flow-cytometry sorted as described above, washed in ice-cold PBS and lysed in lysis buffer (20 mM Tris-HCl (pH 7.5), 150 mM NaCl, 5 mM EDTA (pH 8.0), 5 mM NaPiP, 1 mM, Na 3 VO 4 , 20 mM NaPO 4 (pH 7.6), 3 mM β-glycerophosphate, 10 mM NaF, 1% Triton X-100, complete protease and phosphatase inhibitor cocktail (Roche)) for 15 min on ice. Samples were centrifugated, and whole-cell lysates were collected. Unreduced proteins were separated on a 12% SDS-PAGE, transferred on a nitrocellulose membrane and immunoblotted first with an anti-Phosphotyrosine Ab (Clone 4G10; Millipore) and, after stripping, with an anti-CD3ζ Ab (Clone 6B10.2; Santa Cruz Biotechnology). Signals were quantified using the Image J software. The ratio pζ/ζ was estimated as previously described [54] . Immunofluorescence microscopy Freshly isolated LN cells were first fixed in 4% paraformaldehyde in PBS for 5 min at 37 °C. Ly-6C − and Ly-6C + CD4 T N cells were then sorted using flow cytometry as described above and stained with fluorescein isothiocyanate-conjugated anti-CD4 Ab. T cells were then permeabilized and incubated with an anti-ZAP-70 Ab (Transduction Laboratories) followed by anti-mouse Ab conjugated to Alexa Fluor 647 (Molecular Probes). Stained T cells were photographed on a Yokogawa spinning-disk confocal microscope with a × 100 oil immersion objective connected to a digital video camera and analysed using Image J software. Briefly, automated analysis was performed to divide each cell into quadrants and then to measure the average intensity in each quadrant. The CD4 polarization index was calculated by dividing the highest quadrant by the lowest. Colitis scoring For the colitis model, colons were removed and fixed in PBS containing 10% formaldehyde. Five-micrometer paraffin-embedded sections were cut and stained with haematoxylin and eosin and then blindly analysed. Each segment was given a score of 0–4: grade 0, no significant changes; grade 1, minimal scattered mucosal inflammatory cell infiltrates, with or without minimal epithelial hyperplasia; grade 2, mild scattered to diffuse inflammatory cell infiltrates, sometimes extending into the submucosa and associated with erosions, with mild to moderate epithelial hyperplasia and mild to moderate mucin depletion from goblet cells; grade 3, moderate inflammatory cell infiltrates that were sometimes transmural, with moderate to severe epithelial hyperplasia and mucin depletion; grade 4, marked inflammatory cell infiltrates that were often transmural and associated with crypt abscesses and occasional ulceration, with marked epithelial hyperplasia, mucin depletion and loss of intestinal glands. In vitro polarization assays Flow-cytometry sorted Ly-6C − and Ly-6C + CD4 T N cells from LNs of C57BL/6 Foxp3-GFP mice were stimulated for 4 days with immobilized anti-CD3 (clone 145.2C11; 4 μg ml −1 ; obtained from hybridoma supernatants) and anti-CD28 (clone 37.51; eBioscience; 4 μg ml −1 ) Abs, in the presence of graded concentrations of exogenous recombinant human TGFβ1 (Invitrogen) in the presence (T H 17) or absence (iTreg) of 20 ng ml −1 of recombinant mouse IL-6 (Invitrogen). To study the ability of CD4 T N cells to differentiate into T H 1 effector cells, stimulation was performed in the presence of graded concentrations of recombinant mouse IL-12 (R&D). In vitro suppression assay Purified Ly-6C − or Ly-6C + CD4 T N cells were stimulated for 3 days with coated anti-CD3 and anti-CD28 Abs in the presence of 1 ng ml −1 of TGFβ1 and then let to rest for 3 more days in the presence of recombinant human IL-2 (13 ng ml −1 ; R&D). GFP-expressing cells were then sorted using flow cytometry, and the suppressive capacities of these highly purified Foxp3-expressing cells were then assessed as previously described [31] . Briefly, conventional CD4 T cells (GFP − CD4 + T cells) were purified from LNs of C57BL/6 Foxp3-GFP mice, labelled with Cell Trace Violet (Invitrogen) and stimulated for 64 h, alone or together with Treg cells at various Treg/Tconv-cell ratios. Suboptimal T-cell activation in vitro assay Flow-cytometry sorted Ly-6C − and Ly-6C + CD4 T N cells from LNs of C57BL/6 Foxp3-GFP were stimulated for 3 days with irradiated splenocytes from C57BL/6 CD3ε − / − mice in the presence of graded concentrations of soluble anti-CD3 Ab (145.2C11). These experiments were conducted in the absence of addition of exogenous cytokines. Blocking T-cell entry into LNs C57BL/6 Foxp3-GFP mice were injected or not intraperitoneally with 200 μg of anti-αL and anti-α4 Abs (Bio-Xcell) to block LN entry. Twenty-one hours later, LNs were collected, and CD4 T cells were analysed. In some experiments ( Fig. 6i,j ), 15 × 10 6 T cells from CD45.2 C57BL/6 Foxp3-GFP mice were transferred into C57BL/6 CD45.1 mice lacking (MHC-II − ) or not lacking (MHC-II + ) MHC class II molecule expression. Two hours later, LN entry was blocked as described above. LNs were collected 21 h after entry blockade, and CD45.2 + CD4 T cells were analysed. How to cite this article: Martin, B. et al. Highly self-reactive naive CD4 T cells are prone to differentiate into regulatory T cells. Nat. Commun. 4:2209 doi: 10.1038/ncomms3209 (2013).